Oblique subduction modelling indicates along-trench tectonic transport of sediments Convergent plate margins are currently distinguished as ‘accretional’ or ‘erosional’, depending on the tendency to accumulate sediments, or not, at the trench. Accretion and erosion can coexist along the same margin and we have noticed that this mostly occurs where subduction is oblique. Here we show that at oblique subduction zones, sediments that enter the trench are first buried, and later migrate laterally parallel to the trench and at various depths. Lateral migration of sediments continues until they reach a physical barrier where they begin to accumulate. The accretionary wedge size decreases along the trench moving away from the barrier. We therefore suggest that the gradual variation of the accretionary wedge size and sediment amount at the trench along one single subduction zone, as observed in many active plate margins worldwide, can be explained by the lateral tectonic migration of sediments driven by obliquity of subduction as well. Understanding the nature and dynamics of convergent plate margins is essential to determine the risk related to earthquakes, the petrogenesis in arc settings and the recycling of Earth materials through subduction zones. These particular geodynamic environments have been divided in two main groups: (1) margins dominated by accretion (accretionary margins), where sediments overlaying the subducting plate are stored in a sedimentary prism; and (2) erosive margins, dominated by a long-term landward retreat of the trench that is caused by tectonic removal of fragments from the overriding plate (tectonic erosion); in this case, sediments of the subducting plate are completely buried along with fragments of the overriding margin [1] , [2] , [3] . A slow convergence rate (<7.6 cm yr −1 ) and a thick sedimentary cover of the incoming plate (>1 km) favour accretion of sediments at the trench (case 1). On the other hand, sediments are more efficiently subducted and tectonic erosion is more active when the convergence rate is high (>6 cm yr −1 ) and the sedimentary cover is <1 km (case 2) [2] , [3] , [4] . Long-term tectonic erosion is largely controlled by the episodic collision of large topographic ridges with the trench [2] . A variation in the trench sediment thickness can also be related to a depth gradient developed in the oceanic basement or to the presence of major canyons that allow the deposition of sediments as fans that thicken sediments at the trench floor [5] . It has been observed that in some places, accretion and erosion can coexist along the same margin [6] , [7] , [8] , [9] , [10] , [11] . According to many authors, this heterogeneity is controlled by several parameters, such as the variability in sediment supply to the trench, regulated by contrasting climate (that governs the erosional rate of the arc/fore-arc region) [12] , variable horizontal stress fields (compressional or tensional field) [10] or collision with seamounts that transform an accretionary margin into a short-period erosive margin. [3] , [11] , [13] By analysing the data collected by Heuret et al. [9] and references therein, we have observed that a gradual variation of thickness of the sedimentary prism (from a sediment-starved to a sediment-rich trench) along a single margin mostly occurs where subduction zones are oblique (for example, southern Ryukyu, New Britain, Hikurangi and Sumatra subduction zones), that is, where a trench-normal and a trench-parallel motion of the subducting plate are both present. Here, to test how the trench-parallel motion of the plates could affect geometries and dynamics of sediment subduction and accretion along one single subduction zone, we investigated three-dimensional numerical subduction models (see Methods) in which an oceanic plate sinks obliquely into the mantle. We propose that one of the mechanisms that contribute to the gradual variation of accretionary wedge size observed along several active plate margins could be the lateral tectonic migration of sediments entering the subduction zone coupled with a transport of sediments due to the possible topographic gradient occurring in the trench axis. Reference model development We simulated four different subduction scenarios (see Supplementary Table S1 ) by changing plate convergence rate (3.15–10.95 cm yr −1 ), obliquity of subduction (15–45°) and friction coefficient of sediment (0–0.05). 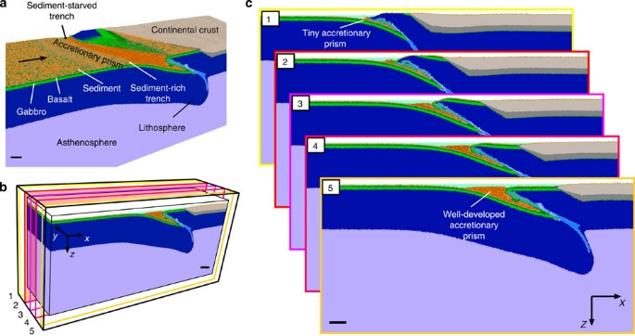Figure 1: Numerical model of an oblique subduction zone. Reference model at 5 Ma after subduction initiation (scale bars, 30 km). (a) Three-dimensional visualization of the subduction zone showing the lateral heterogeneous geometry of the accretionary prism; air and water layers have been graphically removed to show seafloor geometries. (b) Three-dimensional model with the trace of cross-sections. (c) Cross-sections along thex–zplane cut every 50 km alongyaxis. The figure shows the variation in sediments amount both in the accretionary prism and along the subducting slab related to their lateral tectonic migration. Sediments entering the trench migrate from section 1 to sections 2, 3 and 4 following the oblique direction of subduction of the lower plate; in section 5, sediments accumulate because of the model boundary serving as a physical barrier. Figure 1 shows the reference model development for a plate convergence rate of 3.15 cm yr −1 and a continental margin inclined at 45° to the subduction direction. During the simulated subduction process, sediments on top of the incoming oceanic plate are dragged downwards by the subducting slab and a portion of the sediments accumulates at the trench, forming an accretionary prism. However, the oblique motion of the plates at the trench produces a continuous lateral tectonic transport of sediments that move in the direction of the along-trench velocity component of the subducting plate. The lateral migration of sediments is highlighted by the increase in the amount of sediments (both within the subduction channel and in the accretionary prism) in a sequence of sections cross-cutting the trench ( Fig. 1c and Table 1 ) and by the sediment velocity vectors both near the surface and at greater depths ( Supplementary Fig. S2 ). As a consequence of sediment migration, sediment-starved and sediment-rich regions start to form along the trench at the two lateral model boundaries ( Fig. 1a ). During the first million years after subduction initiation, no sedimentary prism forms at the sediment-starved region of the margin; sediments are in fact completely subducted and part of them moves away laterally along the slab; with subduction progress, sediments also start to slowly accumulate at this part of the trench, even if they continue to move laterally. As the lateral boundaries of our models are not permeable to material transit and are stationary, the lateral migration of sediments is blocked at the sediment-rich region close to the model boundary. In our models, this refractory boundary has the role of a physical barrier to the lateral sediment transport, which may exist in natural subduction zones. The accretionary prism near this physical barrier therefore starts to widen with time ( Fig. 2 ) and gradually propagates along the margin in the direction opposite to the lateral sediment transport. Figure 1: Numerical model of an oblique subduction zone. Reference model at 5 Ma after subduction initiation (scale bars, 30 km). ( a ) Three-dimensional visualization of the subduction zone showing the lateral heterogeneous geometry of the accretionary prism; air and water layers have been graphically removed to show seafloor geometries. ( b ) Three-dimensional model with the trace of cross-sections. ( c ) Cross-sections along the x–z plane cut every 50 km along y axis. The figure shows the variation in sediments amount both in the accretionary prism and along the subducting slab related to their lateral tectonic migration. Sediments entering the trench migrate from section 1 to sections 2, 3 and 4 following the oblique direction of subduction of the lower plate; in section 5, sediments accumulate because of the model boundary serving as a physical barrier. Full size image Table 1 Estimate of areas occupied by sediments. 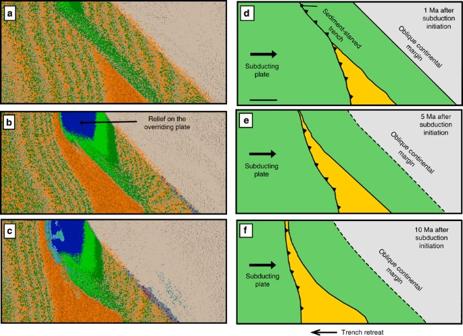Figure 2: Evolution of the accretionary prism with time. The evolving process is represented through the reference numerical model (a,b,c) and schematic sketches (d,e,f). The lines with triangles depict the positions of the trench (triangles are on the overriding plate). Scale bar in (d), 50 km. Full size table Figure 2: Evolution of the accretionary prism with time. The evolving process is represented through the reference numerical model ( a , b , c ) and schematic sketches ( d , e , f ). The lines with triangles depict the positions of the trench (triangles are on the overriding plate). Scale bar in ( d ), 50 km. Full size image Origin and velocity of sediments A portion of the sediment in the accretionary prism derives from the erosion of the relief that forms on the overriding plate as a result of the partial coupling between the lower and upper plates in the sediment-starved region of the trench ( Fig. 2 ); sediment therefore migrates from the highest to the lowest topographic areas and contributes to thickening of the accretionary wedge. Sediments in the accretionary wedge and in the trench therefore derive from both the cover of the incoming oceanic plate and from erosion of the upper plate. The models that we produced do not, however, allow us to discriminate the internal sedimentary structures in the trench and in the accretionary wedge, and hence the structural relationship between them. Sediment migrates laterally with a velocity comparable to the plate convergence rate (1–2 cm yr −1 ) during the first few million years (5 My); velocity increases in the range of 6–12 cm yr −1 (with local peaks of 18 cm yr −1 ) as subduction continues, which could suggest a sort of lateral extrusion along the subducting plate ( Supplementary Fig. S2b ). In the sediment-starved area of the margin, some million years after subduction initiation (5 Ma), sediments stored in the accretionary prism represent around 15–20% of the total amount of sediment that has entered the subduction zone ( Table 1 ). Proceeding along the trench, the percentage of sediment accumulated in the prism increases (from 50 to 70%). With subduction progress, this percentage decreases along the whole margin; sediment is therefore more easily subducted and not stored in the prism. The simulated oblique subduction zone therefore shows a gradual transition from a sediment-starved to a sediment-rich margin ( Fig. 3 ): in the sediment-poor region almost all the incoming sediment is buried at depth, whereas in the sediment-rich part of the margin a well-developed accretionary prism forms. 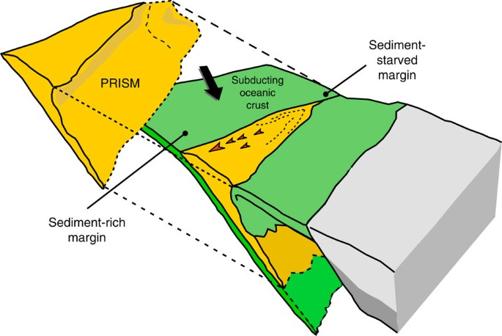Figure 3: Sketch of the heterogeneous geometry of the accretionary prism along a single plate margin. Lateral migration of sediments (red arrows) produces a sediment-starved region along the trench and areas where a wide sedimentary wedge forms. Figure 3: Sketch of the heterogeneous geometry of the accretionary prism along a single plate margin. Lateral migration of sediments (red arrows) produces a sediment-starved region along the trench and areas where a wide sedimentary wedge forms. Full size image Trench rotation and end of sediment migration A 40-My subduction development produces a gradual rotation of the trench that becomes less and less oblique compared with the main convergence vector. The main consequence of this changing geometry is that the lateral tectonic transport of sediment decreases through time according to the lower obliquity of the trench. A difference in sediment amount along the trench persists even after the cessation of sediment lateral tectonic migration, preserving the sediment-starved and sediment-rich sectors along the same trench. In the literature (see above), different convergence rates of plates and different thickness of the sedimentary cover of the incoming oceanic plate along the axis of the trench have so far been considered as the two main factors controlling the heterogeneous sedimentary amount along the same convergent margin. However, in each model that we have run, these two parameters are constant during the whole process and along the trench; therefore, their influence on the sedimentary amount along one single trench can be neglected. Comparisons with the reference model Our additional models ( Supplementary Table S1 ) moreover highlight that greater degrees of obliquity of the subduction zone, or high convergence velocity of the plates, sharpen the along-trench variations in the accretionary prism size. Higher friction coefficient of sediment (0.05) produces only a steeper oceanward slope of the accretionary prism and a trench closer to the continental margin. Our models fit the configuration of several oblique subduction zones worldwide (southern Ryukyu, Hikurangi, Sumatra and New Britain); in fact, these natural examples show a variation of the accretionary prism size along the trench and are, in some way, laterally delimited by lateral physical barriers such as those in our models. Selected natural examples are listed below: at the southern Ryukyu intraoceanic subduction zone ( Fig. 4 ), the Philippine seaplate subducts beneath Eurasia with a right-lateral strike-slip component; thickness of sediments at trench increases from 0.2 km (eastern sector) to 2.5 km (western sector) following the direction of subduction of the Philippine seaplate [9] . Maximum sediment thickness occurs where the trench stops against the Chinese continental margin, the site of collision between the northern Luzon arc and Eurasia [14] , [15] . Moreover, Lallemand et al. [13] noticed that in this area, slip partitioning is either partly accommodated along a transcurrent fault located at the rear of the accretionary prism for obliquity angle of 40° or distributed over the width of the sedimentary wedge when obliquity increases to 60°; the Ryukyu accretionary wedge therefore moves laterally towards Taiwan relative to the Ryukyu Arc [13] . Oblique subduction of the Pacific plate under the Australian continental margin (right-lateral strike-slip component) occurs at the Hikurangi trench ( Fig. 4 ) [16] , [17] . Sediment thickness along the trench varies from 0.8 km (northern sector) to 4.2 km (southern sector) [9] according to the direction of motion of the subducting Pacific plate. This subduction zone is delimited by the continental collision between the Pacific and the Australian plates (South Island of New Zealand) that represents the limit against which the accretionary wedge reaches its maximum size. The Indian/Australian plate sinks obliquely (right-lateral strike-slip component) under the Eurasian plate at the Sumatra subduction zone [18] , [19] ; the thickness of the accretionary wedge increases from 0.9 km (southeastern sector) to 4 km (northwestern sector) [9] following the direction of motion of the subducting plate; the presence of strong curvature of the trench could represent a limit for the lateral migration of sediments that accumulate in this area and increase the size of the accretionary wedge. The New Britain trench has little or no accretionary wedge to the east (thickness of the prism=0.1 km) but the thickness of the accretionary prism increases to the west, reaching 2.5 km (refs 4 , 9 , 10 , 20 ). Subduction of the Solomon Sea plate beneath the South Bismarck plate at the New Britain trench started during the late Miocene or Pliocene [10] , [21] ; at that time, the lower plate was directed northward and the trench was oriented in such a way that a slightly oblique subduction [22] with a right-lateral strike-slip component occurred. The increase in the accretionary prism dimension is therefore consistent with the direction of motion of the Solomon Sea plate compared with that of the upper plate during the first stages of subduction. The accretionary prism and, therefore, the lateral migration of sediments stopped against the collision tip between the Australian continental margin and the Bismarck arc [10] , [20] . 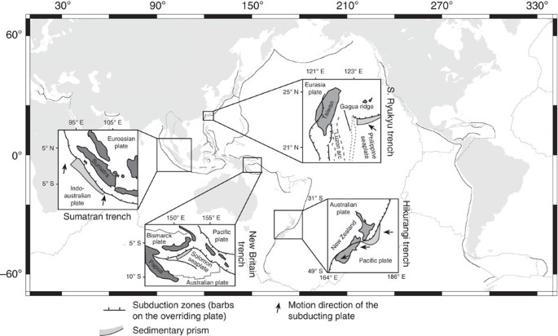Figure 4: World map with the location of the described oblique subduction zones. Modified after Heuretet al.9, the thick black lines (with barbs in the insets) express subduction zones (with barbs on the overriding plate), the thin black lines are ridges; the insets depict each of the trenches we describe in the text (Sumatran, southern Ryukyu, New Britain and Hikurangi), each with a representation of the main regional geological features; arrows indicate motion direction of the subducting plate, the light-grey shaded area represents the sedimentary prism and illustrates its variation in thickness at the trench. Figure 4: World map with the location of the described oblique subduction zones. Modified after Heuret et al. [9] , the thick black lines (with barbs in the insets) express subduction zones (with barbs on the overriding plate), the thin black lines are ridges; the insets depict each of the trenches we describe in the text (Sumatran, southern Ryukyu, New Britain and Hikurangi), each with a representation of the main regional geological features; arrows indicate motion direction of the subducting plate, the light-grey shaded area represents the sedimentary prism and illustrates its variation in thickness at the trench. Full size image All the described subduction zones (with the exception of Sumatra) are relatively ‘young’ (maximum 25 My for the Hikurangi subduction zone (refs 14 , 17 and references therein , 19 )); we therefore think that their general dynamics and geometries can be described by our models. If we consider more mature examples (that is, the Sumatra subduction zone), models can be valid in describing the dynamics acting at the subduction zone as, for example, tectonic lateral migration of sediments. However, geometries in these particular subduction zones can differ from those depicted in the models, as they show only a short range of subduction development (about 40 My). According to the evidence offered from our models, we therefore suggest that lateral tectonic migration of sediments, coupled with the presence of a lateral barrier that stops the trench-parallel motion of sediments, could explain the gradual variation of accretionary wedge size and the transition from a sediment-starved to a sediment-rich trench as observed in many present oblique subduction zones worldwide. As shown in the models, trench sediment thickness can also change with the morphology of the ocean basement (that is, the presence of reliefs or variable plate bending) that produces a gradient in the trench axis; this gradient can partly control the transport of sediment that moves towards the deeper part of basins. We therefore conclude that the gradual variation of accretionary wedge thickness observed along several active plate margins could be explained with the lateral tectonic migration of sediments approaching the subduction zone (testified by the velocity vectors at depth) coupled with a transport of sediments due to the possible topographic gradient occurring in the trench axis. Our models show that in oblique subduction zones, sediment is driven by the trench-parallel motion of the subducting plate and that it moves laterally. However, a gradual variation of accretionary wedge size occurs when a barrier obstructs the lateral transit of sediment and imposes its accumulation. Moreover, we highlight that the differences in accretionary prism size along the trench are emphasized by a greater degree of obliquity of the subduction zone and higher convergence velocities of the plates. As explained in the text, the factors influencing the size of the sedimentary prism are, however, numerous and the lateral motion of sediments is only one of the mechanisms acting at oblique subduction zones that possibly shape accretionary prisms. Furthermore, we are aware that models remain limited in their ability to fully describe the natural systems and their complexity. In this study, we therefore give only a suggestion regarding possible sediment behaviour at oblique subduction zones that could help interpret field and geophysical data to better understand active plate margin dynamics. Initial model setup The models are solved using I3ELVIS code; it is based on the numerical solution of mass, momentum and energy conservation equations using finite difference method and marker-in cell techniques combined with a multigrid solver [23] , [24] . The staggered grid for which equations are solved includes 501 × 165 × 101 nodes with 100 million randomly distributed markers. The initial model setup simulates a 1,000-km-long, 328-km-high and 200-km-wide box in which an infinite wide oceanic basin delimited by a continental margin is reproduced ( Supplementary Fig. S1 ). The oceanic basin is floored by a layered oceanic crust where a 5-km-thick layer of gabbro is overlain by a 3-km-thick layer of basalt. The sequence is sealed by a 1-km-thick cover of sediments. Sediments extend for a few kilometres on the continental margin as well. The represented oceanic basin has a homogeneous age of 30 Ma. The subduction is prescribed to start at a weak zone (20 km thick and 75 km deep) in the mantle (wet olivine rheology, brittle/plastic strength 1 MPa), located 100 km seaward from the continental margin. The weak zone represents the decoupling area between the two plates and it virtually corresponds to a shear zone that dips in the mantle. The dip angle of the weak zone ( Supplementary Table S1 ) controls the initial inclination of the subducting plate that evolves with time. A homogeneous plate velocity is applied on both lateral sides of the model ( Supplementary Table S1 and Supplementary Fig. S1 ) to simulate convergence of the plates. In the reference model (cmbl), the plate at the ‘right’ side has a velocity of 0.95 cm yr −1 , whereas the plate at the ‘left’ side moves with a velocity of 2.2 cm yr −1 . The ‘obliquity’ of subduction varies accordingly to the angle between the trace of the weak zone (that is the place of subduction initiation) on the horizontal plane and the lateral boundaries of the model to which convergence velocity is applied ( Supplementary Table S1 and Supplementary Fig. S1 ). Rock rheology and boundaries conditions Visco-plastic rock rheology is described by experimentally determined flow laws [25] , in which the effective viscosity η creep is a function of temperature, pressure and strain rate ( Supplementary Table S2 ). Serpentinite is described by a weak Newtonian rheology with the constant viscosity of 10 18 Pa s (ref. 26 ). Low-viscosity and -density air and water layers (density=1 kg m −3 , viscosity=10 19 Pa s) and sea water (density=1,000 kg m −3 , viscosity=10 19 Pa s) at the top of the model simulate a free-surface-like condition for the crust; the solid portion of the model thus behaves as a free erosion/sedimentation surface [27] . Erosion and sedimentation are implemented in a highly simplified manner: sea level is set at 12 km from the top of the model, positive topography >4 km above the sea level is instantaneously eroded, trench is instantaneously filled by sediments at depths >8 km below the sea level. All model boundaries are free slip, except for the lower one that is permeable. More detailed information about numerical modelling approach and material properties are given in Zhu et al. [28] and Supplementary Table S2 . An oceanic geotherm [29] defines the initial temperature field of the oceanic plates. A particular geotherm characterizes the temperature field of the transitional zones between the ocean and the continental margins. Fluids and melts After subduction initiation, fluids inside rock porosities or fixed in hydrous minerals are released by the subducting slab; they migrate upward and hydrate the overlying mantle wedge [26] , [30] , [31] , [32] , [33] . Free fluid present in sediments and basalts makes up to 2 wt% at the surface and is believed to decrease with depth. To account for compaction, it is supposed that this water is released, decreasing from 2 wt% to 0 wt% at 75 km depth [34] : where X H2O (p0) =2 wt% is the connate water content at the surface, and Δz is depth below the surface in kilometres (0–75 km). Slab mantle dehydration/hydration algorithm is based on water markers and is similar to previously published subduction models [27] , [30] , [34] . The dehydration reactions that allow H 2 O release by a rock marker are controlled by the physicochemical conditions in the model and by the assumption of thermodynamic equilibrium. The generated water marker includes a particular amount of water and starts to move independently with time until it reaches a lithology that can assimilate H 2 O (ref. 34 ). The local kinematical transport condition gives the velocity of fluid markers as follows [30] : where v x and v z are the local velocity of the mantle and v z (percolation) is the prescribed relative velocity of upward percolation of H 2 O through the mantle. The maximum water content of the mantle wedge hydrated by the slab fluids is 2 wt% (ref. 34 ). The boundary between serpentinite-rich (density=3,000 kg m −3 ) and hydrated serpentinite-free mantle rocks (density=3,300 kg m −3 ) is defined by the stability field of antigorite [33] . Melt is extracted from partially molten rocks considering a melt extraction threshold M max and a non-extractable amount of melt M min < M max that remains in the rock [27] . The amount of melt extracted during subduction is traced by markers. In the models, a constant M max =4 vol% and M max /M min =2 ratio is used. The total amount of melt migrating upward is calculated as reported in Nikolaeva et al. [27] As the velocity of the melt is thought to be rapid compared with the deformation of the unmolten mantle and be unaffected from its dynamics, the extracted melt is instantaneously driven to the surface [27] . How to cite this article: Malatesta, C. et al. Oblique subduction modelling indicates along-trench tectonic transport of sediments. Nat. Commun. 4:2456 doi: 10.1038/ncomms3456 (2013).